Photoautotrophic hydrogen production by eukaryotic microalgae under aerobic conditions Eukaryotic algae and cyanobacteria produce hydrogen under anaerobic and limited aerobic conditions. Here we show that novel microalgal strains ( Chlorella vulgaris YSL01 and YSL16) upregulate the expression of the hydrogenase gene ( HYDA ) and simultaneously produce hydrogen through photosynthesis, using CO 2 as the sole source of carbon under aerobic conditions with continuous illumination. We employ dissolved oxygen regimes that represent natural aquatic conditions for microalgae. The experimental expression of HYDA and the specific activity of hydrogenase demonstrate that C. vulgaris YSL01 and YSL16 enzymatically produce hydrogen, even under atmospheric conditions, which was previously considered infeasible. Photoautotrophic H 2 production has important implications for assessing ecological and algae-based photolysis. Microalgae are microorganisms that use solar energy to combine water with carbon dioxide to create biomass [1] , [2] . The growth kinetics of photoautotrophic algae depend on the extent of available carbon sources (for example, bicarbonate), which are mainly generated from the dissolution of atmospheric carbon dioxide [3] , [4] , [5] , [6] . The common photosynthetic process in algae results in the splitting of H 2 O and the resultant O 2 evolution (driven by light absorbed by photosystem II). Subsequently, electrons are transferred from photosystem I reaction centres to hydrogenase (H 2 ase) through ferredoxin, which is the natural electron donor (driven by light absorbed by photosystem I), while forming biomass or producing energy [7] , [8] , [9] . Under special conditions (anaerobic conditions plus light), photosynthetic electrons are delivered to [FeFe]-H 2 ase instead of NADPH via ferredoxin, and [FeFe]-H 2 ase utilizes them to reduce protons to molecular hydrogen. This reaction is catalysed by [FeFe]-H 2 ase, which is extremely sensitive to oxygen and does not require any extra energy in the form of ATP [10] . In the meantime, cyanobacteria may produce hydrogen either as a by-product of nitrogen fixation using nitrogenase [11] or by a reversible NAD(P)H-dependent NiFe-H 2 ase [12] . Certain unicellular green algae have been well established to be capable of hydrogen metabolism, as has been observed in many taxonomically diverse species, through a variety of biochemical mechanisms and processes with physiological adaptations [13] , [14] . Green microalgae, such as Chlamydomonas reinhardtii , C. noctigama , C. moewusii and Chlorella fusca , synthesize [FeFe]-H 2 ase that is highly active in hydrogen evolution [15] . However, owing to the oxygen sensitivity of [FeFe]-H 2 ases, most studies on photosynthetic hydrogen production have largely relied on experimental manipulations, including intermittent illumination and/or anaerobic conditions [2] , [16] (for example, dissolved oxygen was completely removed from the culture media). A review of previous studies revealed that there are no reports on the occurrence of photoautotrophic H 2 production in the presence of CO 2 and O 2 . Here we show that eukaryotic green algal strains can produce H 2 during inorganic carbon uptake under high O 2 levels that are known to inhibit H 2 ase synthesis and activity. Two eukaryotic microalgal strains, C. vulgaris YSL01 and YSL16, directly produce gaseous hydrogen through photosynthesis under different dissolved oxygen regimes and continuous illumination, using CO 2 as the sole carbon source. The identification of eukaryotic and oxygenic photoautotrophs that can produce hydrogen even under aerobic conditions has important implications for biohydrogen production. Microalgae can produce hydrogen under aerobic conditions Photoautotrophic hydrogen production by C. vulgaris YSL01 increased from 0.3 to 0.6 ml l −1 in 3 days as headspace CO 2 increased from 5 to 15% at 15% O 2 . C. vulgaris YSL16 produced 0.1 ml l −1 of photoautotrophic hydrogen in 4 days under 5% CO 2 and 15% O 2 conditions, and increasing CO 2 to 15% with 15% O 2 improved the hydrogen production to 0.3 ml l −1 in 5 days ( Fig. 1a and Supplementary Fig. 1 ). Under 5% O 2 and 10% CO 2 , C. vulgaris YSL01 and YSL16 produced 1.9 and 1.2 ml l −1 hydrogen in 3 and 4 days, respectively, and increasing the O 2 concentration to 15% with 10% CO 2 decreased hydrogen production to 1.2 and 0.6 ml l −1 for 3 and 4 days of cultivation, respectively ( Fig. 1b and Supplementary Fig. 1 ). The biomass-normalized hydrogen production (ml of H 2 per g of biomass) was similar for elevating headspace CO 2 ( Fig. 1c ), but it significantly decreased from 1.8±0.01 and 1.1±0.03 to 0.6±0.02 and 0.3±0.01 ml g −1 ( P <0.0001), with the elevation of O 2 levels from 5 to 15% at 10% CO 2 for YSL01 and YSL16, respectively ( Fig. 1d ). We used the one way ANOVA test within the GraphPad Prism5 software to generate all P -values. Hydrogen production was even observed in the control atmospheric CO 2 and O 2 condition. Cumulative hydrogen production was relatively higher for C. vulgaris YSL01 compared with YSL16 ( Fig. 1 ). The produced and accumulated hydrogen decreased in response to increasing oxygen content in the headspace, and it was completely removed within 7 days after hydrogen production peaked ( Fig. 2 and Supplementary Fig. 1 ). No further hydrogen production was observed at very high partial pressures of oxygen for both C. vulgaris YSL01 and YSL16. An analogous observation was previously reported, in which hydrogen was consumed by photoheterotrophic eukaryotes under the dark/light anaerobic conditions [2] , [4] . 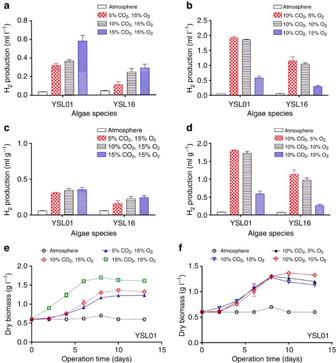Figure 1: Net photoautotrophic hydrogen production by microalgae. Hydrogen produced by algae accumulated in the headspace of serum bottles under various cultivation conditions. (a,b) The amount of hydrogen in the headspace was monitored throughout the cultivation period, and the highest net hydrogen peak (observed at 3, 4 or 5 days of cultivation) for each culture is shown. The highest level of hydrogen production was achieved byC. vulgarisYSL01 (up to 1.9 ml of H2l−1with 5% O2at 10% CO2). (c,d) Biomass-normalized hydrogen production was similar for increasing CO2concentrations from 5 to 15% at 15% O2, whereas it significantly decreased with increasing O2concentrations from 5 to 15% at 10% CO2. (e) The initial biomass concentration ofC. vulgarisYSL01 was 0.6 g dry weight l−1, and this value varied from 0.6 to 1.7 g dry weight l−1after 8 days of cultivation at different initial CO2concentrations ranging from 0.003 (atmospheric) to 15%. (f)C. vulgarisYSL01 had a similar growth rate, with different initial O2levels ranging from 5 to 15% at 10% CO2. For all of the cultivation conditions, the suspension pH in the culture bottles increased from 7.9 (initial) up to 8.7 (end of incubation). Each data point represents the average of triplicate experiments and the ±s.d. Figure 1: Net photoautotrophic hydrogen production by microalgae. Hydrogen produced by algae accumulated in the headspace of serum bottles under various cultivation conditions. ( a , b ) The amount of hydrogen in the headspace was monitored throughout the cultivation period, and the highest net hydrogen peak (observed at 3, 4 or 5 days of cultivation) for each culture is shown. The highest level of hydrogen production was achieved by C. vulgaris YSL01 (up to 1.9 ml of H 2 l −1 with 5% O 2 at 10% CO 2 ). ( c , d ) Biomass-normalized hydrogen production was similar for increasing CO 2 concentrations from 5 to 15% at 15% O 2 , whereas it significantly decreased with increasing O 2 concentrations from 5 to 15% at 10% CO 2 . ( e ) The initial biomass concentration of C. vulgaris YSL01 was 0.6 g dry weight l −1 , and this value varied from 0.6 to 1.7 g dry weight l −1 after 8 days of cultivation at different initial CO 2 concentrations ranging from 0.003 (atmospheric) to 15%. ( f ) C. vulgaris YSL01 had a similar growth rate, with different initial O 2 levels ranging from 5 to 15% at 10% CO 2 . For all of the cultivation conditions, the suspension pH in the culture bottles increased from 7.9 (initial) up to 8.7 (end of incubation). Each data point represents the average of triplicate experiments and the ±s.d. 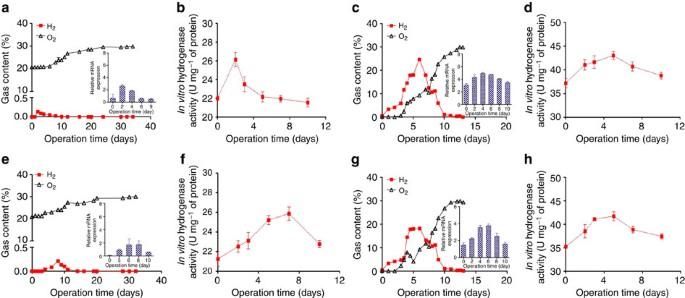Figure 2: Photosynthetic hydrogen production and oxygen evolution. Quantification of the H2ase mRNA synthesized by (a–d)C. vulgarisYSL01 and (e–h)C. vulgarisYSL16 during photoautotrophic cultivation under atmospheric and anaerobic conditions. The kinetics of hydrogen production by two different microalgal isolates was monitored for up to 34 days under (a,e) atmospheric and CO2-limited (closed system) as well as (c,g) anaerobic, 10% CO2, and photoautotrophic conditions using crimp-sealed culture bottles. The highest hydrogen content achieved byC. vulgarisYSL01 and YSL16 under atmospheric condition was 0.17 and 0.23%, whereas under the anaerobic condition at 10% CO2, maximum hydrogen contents of 24.6 and 18.2% were achieved, respectively. (b,f) During the period of aerobic hydrogen production, both normalizedHYDAexpression level andin vitroH2ase activity were quantitatively determined.HYDAwas expressed at various concentrations of oxygen, and its relative mRNA concentration displayed a linear correlation with H2ase activity.In vitroH2ase activity was significantly decreased as the oxygen levels increased (≥21%;P<0.05). (d,h) Under anaerobic conditions, H2ase activity and mRNA expression peaked after 4–6 days of cultivation and then dropped significantly owing to the gradual accumulation of oxygen. The value at each time point represents the average of three independent experiments±s.e. The size of the error bars is smaller than the symbol size. Full size image Figure 2: Photosynthetic hydrogen production and oxygen evolution. Quantification of the H 2 ase mRNA synthesized by ( a – d ) C. vulgaris YSL01 and ( e – h ) C. vulgaris YSL16 during photoautotrophic cultivation under atmospheric and anaerobic conditions. The kinetics of hydrogen production by two different microalgal isolates was monitored for up to 34 days under ( a , e ) atmospheric and CO 2 -limited (closed system) as well as ( c , g ) anaerobic, 10% CO 2 , and photoautotrophic conditions using crimp-sealed culture bottles. The highest hydrogen content achieved by C. vulgaris YSL01 and YSL16 under atmospheric condition was 0.17 and 0.23%, whereas under the anaerobic condition at 10% CO 2 , maximum hydrogen contents of 24.6 and 18.2% were achieved, respectively. ( b , f ) During the period of aerobic hydrogen production, both normalized HYDA expression level and in vitro H 2 ase activity were quantitatively determined. HYDA was expressed at various concentrations of oxygen, and its relative mRNA concentration displayed a linear correlation with H 2 ase activity. In vitro H 2 ase activity was significantly decreased as the oxygen levels increased (≥21%; P <0.05). ( d , h ) Under anaerobic conditions, H 2 ase activity and mRNA expression peaked after 4–6 days of cultivation and then dropped significantly owing to the gradual accumulation of oxygen. The value at each time point represents the average of three independent experiments±s.e. The size of the error bars is smaller than the symbol size. Full size image Increasing the headspace CO 2 improved the biomass production from 1.2 to 1.7 g l −1 , whereas increasing the O 2 level had no profound effect on biomass production ( Fig. 1e,f ). Continuous illumination for the cultivation of these microalgal species resulted in relatively faster growth rates compared with previous studies employing dark/light cycles [17] , [18] . The microalgal growth under continuous illumination was mainly dependent on CO 2 , with little dependence on O 2 . C . vulgaris YSL01 and YSL16 showed the maximum growth rate of 0.11 and 0.08 per day at 15% CO 2 under the investigated experimental conditions ( Fig. 1 and Supplementary Fig. 2 ). Hydrogen production at high oxygen concentration The H 2 ase gene ( HYDA ) was expressed and detected even at high concentrations of oxygen (≥21%, initially atmospheric condition), and its relative concentration showed a linear correlation ( R 2 =0.94 and 0.63 for YSL01 and YSL16, respectively) with photosynthetic hydrogen production under the given experimental conditions ( Fig. 2a,c ). In vitro H 2 ase activity also supported the changes in hydrogen production ( Fig. 2b,d and Supplementary Fig. 3 ). These results are indicative of the oxygen tolerance of H 2 ase in the algal cells exposed to high oxygen concentrations for a long period of time. The headspace hydrogen reached a maximum concentration of 0.15–0.69% within 7 days of cultivation for both algal species ( Supplementary Fig. 1 ). Under anaerobic conditions, higher H 2 ase activity and messenger RNA expression resulted in significantly more hydrogen production compared with the atmospheric environment. The H 2 ase activity of YSL01 reached a maximum (43.86±1.68 U mg −1 of protein; P <0.05) after 5 days of cultivation, which correlated with the mRNA expression and hydrogen production. An increase in the headspace O 2 concentration (>10%) due to microalgal photosynthetic activity decreased the H 2 ase activity and hydrogen production ( Fig. 2c,g ). 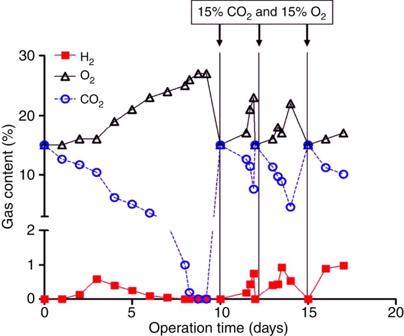Figure 3: Hydrogen production and consumption byC. vulgarisYSL01. The headspace was recirculated at intervals with a gas mixture composed of 15% O2, 15% CO2and 70% N2, and photoautotrophic hydrogen production was monitored throughout the 18-day cultivation period. Hydrogen production ceased and the sequential consumption of the accumulated hydrogen occurred when the oxygen level in the headspace exceeded the critical oxygen concentration. Individual data points represent the average of two independent experiments. Figure 3 shows the microalgal hydrogen production and consumption under CO 2 -enriched aerobic conditions in response to the variations in the headspace oxygen levels, which varied from 15 to 26% as a result of photosynthetic O 2 production. Hydrogen production ceased and the subsequent consumption of the accumulated hydrogen occurred when the oxygen level in the headspace exceeded the critical O 2 concentration (that is, >21% O 2 ). The headspace was flushed at intervals with a gas mixture containing 15% O 2 , 15% CO 2 and 70% N 2 , and a similar trend was observed regarding the fate of hydrogen in the headspace. To ascertain whether the H 2 ase was reactivated or resynthesized, we quantified H 2 ase activity and mRNA expression at 10 days when hydrogen production had ceased. The H 2 ase activity and mRNA expression decreased to a value similar to those of day 0 ( Fig. 2 ), suggesting that the hydrogen production observed after flushing the headspace with the gas mixture might be because of the reactivation of H 2 ase, which was inactivated above the critical concentration of oxygen ( Fig. 3 ). The potential reactivation of this enzyme was demonstrated by determining the specific H 2 ase activity in the algal cells grown under anaerobic conditions, followed by their subsequent exposure to aerobic and anaerobic environments. The exposure to aerobic conditions inhibited H 2 ase activity by 72.5%, but the subsequent exposure to anaerobic conditions reactivated the H 2 ase, restoring 73% of the initial specific H 2 ase activity ( Supplementary Table 1 ). Notably, H 2 ase was reactivated even after exposure to 25% O 2 for more than 48 h ( Fig. 3 ). Figure 3: Hydrogen production and consumption by C. vulgaris YSL01. The headspace was recirculated at intervals with a gas mixture composed of 15% O 2 , 15% CO 2 and 70% N 2 , and photoautotrophic hydrogen production was monitored throughout the 18-day cultivation period. Hydrogen production ceased and the sequential consumption of the accumulated hydrogen occurred when the oxygen level in the headspace exceeded the critical oxygen concentration. Individual data points represent the average of two independent experiments. Full size image H 2 ase activity correlates with initial oxygen levels In vitro H 2 ase activity in both microalgal strains cultivated under various headspace oxygen levels was determined after replenishment with oxygen-free nitrogen for 5 min to activate the H 2 ase under strictly anaerobic conditions. A decrease in the specific H 2 ase activity and in vitro H 2 ase activity was observed for both microalgal species with increasing initial headspace O 2 , indicating that H 2 ase activity was strongly influenced by the amount of oxygen ( Fig. 4 and Supplementary Fig. 3 ). These data support the significant decrease in hydrogen production with higher initial O 2 concentration ( Fig. 1b,d ). Relatively higher H 2 ase activity was observed under lower initial O 2 conditions (5–10%) compared with the higher O 2 environment (atmospheric O 2 ), but no apparent correlation was observed between the specific H 2 ase activity and the microalgal biomass amount as the activity significantly varied for similar biomass when the inorganic carbon concentration was fixed at 10% ( Figs 1f and 4 ). H 2 ase is extremely sensitive to oxygen, and its activity is inhibited even on exposure to low concentrations of oxygen [19] . However, in the present study, H 2 ase activity at partial pressure of oxygen (5–21%) consistently indicated that the microalgae could perform hydrogen production and/or H 2 ase synthesis, even in 21% oxygen ( Figs 2 and 4 and Supplementary Fig. 3 ). 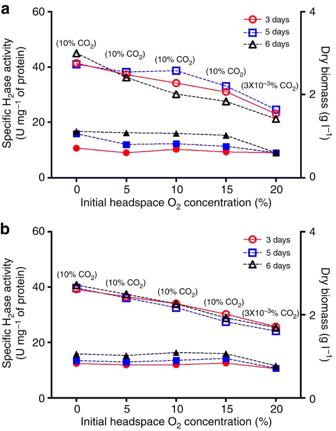Figure 4: Specific activity of H2ase in microalgal dry biomass. The specific activity of H2ase (empty symbols) in (a)C. vulgarisYSL01 and (b)C. vulgarisYSL16 cultured under different O2levels in the headspace at 3, 5 and 6 days of cultivation was determined after flushing the microalgal biomass (filled symbols) with oxygen-free nitrogen gas for 5 min to activate H2ase under strictly anaerobic conditions. The specific activity of H2ase decreased with increasing initial O2in the headspace for the investigated microalgal species, indicating that the enzyme activity was strongly influenced by the amount of oxygen. The numbers in parentheses represent the initial CO2concentrations. Individual data points represent the average of two independent experiments. Figure 4: Specific activity of H 2 ase in microalgal dry biomass. The specific activity of H 2 ase (empty symbols) in ( a ) C. vulgaris YSL01 and ( b ) C. vulgaris YSL16 cultured under different O 2 levels in the headspace at 3, 5 and 6 days of cultivation was determined after flushing the microalgal biomass (filled symbols) with oxygen-free nitrogen gas for 5 min to activate H 2 ase under strictly anaerobic conditions. The specific activity of H 2 ase decreased with increasing initial O 2 in the headspace for the investigated microalgal species, indicating that the enzyme activity was strongly influenced by the amount of oxygen. The numbers in parentheses represent the initial CO 2 concentrations. Individual data points represent the average of two independent experiments. Full size image This study demonstrates that two novel microalgal strains ( C. vulgaris YSL01 and YSL16) are capable of photoautotrophic hydrogen production during exposure to continuous illumination under aerobic conditions. Photosynthesis in these photoautotrophic green algae directly produced gaseous hydrogen under aerobic conditions. The amount of hydrogen produced was different for YSL01 and YSL16. Photoautotrophic hydrogen production was significantly increased when the algae grew under high CO 2 conditions but the biomass-normalized hydrogen production demonstrated a limited effect in response to CO 2 elevation, indicating that the increase in biomass production due to CO 2 elevation enhanced photoautotrophic hydrogen production. The elevation of headspace O 2 significantly decreased hydrogen production. The H 2 ase in these microalgae may be tolerant to high levels of oxygen and, thus, the activity of H 2 ase was not completely inhibited even in the presence of atmospheric oxygen levels. Potential H 2 ase reactivation was also observed after the exposure to 25% headspace oxygen for 48 h. Photosynthetic organisms were previously reported to display a slow rate of H 2 production owing to the oxygen sensitivity of H 2 ase [20] , [21] . Thus, the sensitivity of H 2 ase to oxygen has been implicated as a major obstacle to improving phototrophic biological hydrogen production [22] . However, Chader et al. [23] showed that Chlorella sp. (eukaryotic microalga) produced small amounts of hydrogen with O 2 partial pressure up to 15% in the headspace under mixotrophic conditions. Here we showed that novel microalgal strains ( C. vulgaris YSL01 and YSL16) can produce hydrogen through photosynthesis using CO 2 as the sole source of carbon with continuous illumination under aerobic conditions. The amount of hydrogen produced was strongly influenced by the initial oxygen concentration. The identification of photoautotrophic hydrogen production by eukaryotic algae under different oxygen levels (including atmospheric conditions) is ecologically important as the massive growth of algae can change the local environmental conditions in terms of H 2 bioavailability in the natural aquatic system below the water surface, resulting in different oxygen regimes. The relative expression of HYDA mRNA and the specific activity of H 2 ase revealed that hydrogen production was facilitated by H 2 ase expression under atmospheric oxygen levels. This study provides evidence of a naturally evolved oxygen-tolerant H 2 ase in eukaryotic microalgae, and further study may open a new avenue for continuous biophotolysis to produce hydrogen and an opportunity to develop an artificial oxygen-tolerant H 2 ase-based biomimetic photovoltaic cell using eukaryotic algae. Strain isolation and growth conditions C. vulgaris strains (YSL01 and YSL16) were isolated from a local lake, Wonju, South Korea ( Supplementary Fig. 4 and Supplementary Table 2 ). Subcultures were made by inoculating Petri plates containing EDTANa 2 -lacking bold basal medium (BBM) solidified with 1.5% (w/v) bacteriological agar with 50 μl of culture solution. In addition, 50 μl aliquots of the same dilutions were plated in 96-well microtiter plates containing 200 μl of EDTANa 2 -lacking BBM. The purity of the culture was confirmed by repeated plating and by regular observation using a microscope. Each microalgal species, with an initial optical density of 0.3–0.5 at 680 nm, was inoculated into 500 ml aluminium crimp-sealed culture bottles containing 250 ml of EDTANa 2 -lacking BBM. The experiments were performed in triplicate using 500 ml culture bottles with a working volume of 250 ml. The experimental bottles were incubated under white fluorescent light with an illumination of 50 μmol m −2 s −1 at 27 °C for 5 weeks with shaking at 150 r.p.m. and without organic carbon supplementation. The headspace of the culture bottles was artificially replaced with four different gas mixtures comprising N 2 , CO 2 and O 2 . The initial partial pressures of both CO 2 and O 2 ranged from 5 to 15%, and atmospheric conditions were also investigated. The specific growth rate (μ) was calculated as described by Jiang et al. [24] Hydrogen and oxygen measurements H 2 and O 2 in the headspace of the serum bottles was periodically measured using a GC-14 gas chromatograph (Shimadzu, Kyoto, Japan) equipped with a thermal conductivity detector and a molecular sieve 5A 80/100 column, using Ar as a carrier gas. Crude cell extract and H 2 ase activity The crude cell extract preparation and the measurement of H 2 ase activity were performed as described by Ueno et al. [25] In brief, microalgae cultivated under the different O 2 concentrations for 0–8 days were harvested at regular time intervals by centrifugation (12,000 g , 4 °C, 15 min) and washed twice in 20 mM phosphate buffered (pH 7.5) 1% NaCl solution. The resulting pellet was resuspended in an equal volume of the same buffer, and the cell suspension was flushed with oxygen-free nitrogen gas under anaerobic conditions. After 5 min (or 24 h, which is only for the experimental results in Supplementary Table 1 ) of anaerobic adaptation, the cells were harvested by centrifugation (12,000 g , 4 °C, 20 min) and resuspended in a basal buffer containing 50 mM Tris (hydroxymethyl) aminomethane–HCl (pH 8.0), 2 mM MgCl 2 and 1 mM dithiothreitol, followed by the addition of powdered sodium dithionite (50 mM). The suspension was placed in a sealed steel beaker, sonicated at 300 W for 10 min in an ice-water bath under a pulsed 75%-duty-cycle condition (Sonomasher, Ulsso-Tech, Seoul, Korea) and centrifuged at 15,000 g for 20 min at 4 °C. The crude extract was prepared under strict anaerobic conditions at 4 °C. H 2 ase activity was quantified by the amount of hydrogen evolved from methyl viologen, which was reduced by sodium dithionite. Hydrogen production was determined by gas chromatography using a thermal conductivity detector (GC6890A, Agilent Technologies, Santa Clara, CA, USA). The assays were prepared in seal-lock vials (20 ml) with equal volumes of the liquid and gas phases. The sample (0.1–0.25 ml) was injected into 10 ml of basal buffer containing 5 mM methyl viologen and 5 mM sodium dithionite and incubated in a shaker at 28 °C for 30 min. One unit of activity was defined as the amount of H 2 ase needed to evolve 1 μmol of hydrogen gas per minute. The protein concentration in the crude extracts was determined by the Bradford method using BSA as a standard. Total RNA isolation and H 2 ase gene detection Total RNA was isolated from the algal cells using the RNeasy kit (Qiagen, Valencia, CA), according to the manufacturer’s instructions [26] . mRNA was harvested from microalgae cultivated under different O 2 concentrations for 8 days. The RNA concentration of each sample was determined by measuring the absorbance at 260 nm using a spectrophotometer. The integrity of each RNA sample was evaluated using the Agilent 2100 BioAnalyzer (Agilent Technologies). Complementary DNA synthesis was performed with 1 μg of total RNA using random primers (Invitrogen, Carlsbad, CA) and Superscript II reverse transcriptase (Invitrogen). Real-time reverse transcriptase PCR analyses were performed using a 7500 Real-Time PCR System (Applied Biosystems Inc, Foster City, CA). Reactions were performed in a 25-μl volume containing 12.5 μl of 2X SYBR Green reaction buffer, 1 μl of cDNA (corresponding to 25 ng of reverse transcribed total RNA) and 5 pmol of each HYDA -specific primer obtained from C. fusca (GenBank accession number AJ298228 ). After an initial incubation for 2 min at 50 °C, the cDNA was denatured at 95 °C for 10 min, followed by 45 cycles of PCR (95 °C for 15 s and 60 °C for 60 s). The data analyses were performed using 7500 system SDS software, version 1.3.1 (Applied Biosystems Inc). For the time course experiment, the samples were collected during hydrogen production, starting from 0 time under atmospheric conditions. The relative HYDA expression levels for all samples were calculated and normalized with respect to the 18S ribosomal RNA expression levels. The following primers were used: HYDA (AJ298228.1) forward, 5′-TGTCCTCCAACACCTCAGGC-3′; HYDA reverse, 5′-CTCCTGCTCTCCTTGGGCTT-3′; 18S rRNA (DQ644506.1) forward, 5′-GGCTTAATTGTCCGGGACTC-3′; and 18S rRNA reverse, 5′-AATGAAATACGAATGCCCCC-3′. How to cite this article: Hwang, J.-H. et al. Photoautotrophic hydrogen production by eukaryotic microalgae under aerobic conditions. Nat. Commun. 5:3234 doi: 10.1038/ncomms4234 (2014).